A protein phosphatase 2A complex spatially controls plant cell division In the absence of cell migration, the orientation of cell divisions is crucial for body plan determination in plants. The position of the division plane in plant cells is set up premitotically via a transient cytoskeletal array, the preprophase band, which precisely delineates the cortical plane of division. Here we describe a protein complex that targets protein phosphatase 2A activity to microtubules, regulating the transition from the interphase to the premitotic microtubule array. This complex, which comprises TONNEAU1 and a PP2A heterotrimeric holoenzyme with FASS as regulatory subunit, is recruited to the cytoskeleton via the TONNEAU1-recruiting motif family of proteins. Despite the acentrosomal nature of plant cells, all members of this complex share similarity with animal centrosomal proteins involved in ciliary and centriolar/centrosomal functions, revealing an evolutionary link between the cortical cytoskeleton of plant cells and microtubule organizers in other eukaryotes. Fine-tuning of the spatial positioning of division planes is crucial for coordinating multicellular development in plants [1] , [2] . Cells of land plants are glued together by a pecto-cellulosic cell wall, and do not have the ability to migrate. Their location is set up irreversibly by oriented cell divisions occurring in specialized histogenic tissues, the meristems. Consequently, the three-dimensional cellular organization of a plant tissue closely reflects the pattern of cell division and cell expansion that has occurred during its development. In contrast to animal cells, plant cells establish their plane of division early during the cell cycle, and one of the first conspicuous signs of commitment to division is the transition of the cortical microtubular array into a dense preprophase band (PPB) encircling the nucleus [3] . The PPB precisely forecasts the cortical region reached by the growing cell plate during cytokinesis. It is thus supposed to leave a positional cue at the cell cortex, which persists there until cytokinesis [2] , [4] . At the end of prophase, the PPB disappears concomitantly with nuclear envelope breakdown and spindle formation. In telophase, the new cell plate separating the daughter cells is deposited through vesicle transport guided by a mitotic cytoskeletal array composed of actin filaments and microtubules, the phragmoplast, which initiates at the centre of the cell, and grows centrifugally until it connects with the plasma membrane at the cortical site previously occupied by the PPB. Thereafter, microtubules re-colonize the cell cortex and organize into parallel arrays transverse to the cell elongation axis, guiding deposition of cellulose microfibrils on the outer side of the cell [5] , [6] . Unlike many eukaryotes, cells of land plants lack a conspicuous microtubule organizing centre (MTOC) such as a centrosome, with the exception of basal bodies formed briefly in flagellate motile sperm cells of land plants that rely on aqueous fertilization (mosses and ferns). Siphonogamous Angiosperms and Pinophytes are devoid of centrosomes and centrioles at any stage. Few genes involved in PPB formation have been identified [7] . Among them, TON1 and FASS / TON2 are the only ones whose disruption leads to a complete absence of PPB formation. Arabidopsis mutants in either TON1 or FASS display identical phenotypes [8] , [9] , [10] , [11] , [12] : plants are dwarf and misshapen, display abnormal cell elongation and random positioning of cell division planes [8] , [9] . In addition to absence of PPBs in premitotic cells, interphase microtubule arrays are also affected, and lack the typical parallel organization of wild-type cells [9] , [10] , [11] . In maize, simultaneous loss of function of the two FASS homologues is embryo lethal, while TON1 disruption in moss phenocopies the developmental syndrome of Arabidopsis ton1 mutants [13] , [14] . The TON1 N-terminus shares sequence similarity with the animal centrosomal proteins FOP and OFD1 and interact with Arabidopsis CENTRIN [11] , which in animal cells is a major constituent of MTOCs. TON1 has recently been shown to interact with TON1-recruiting motif proteins (TRMs) [15] , which possess several motifs also present in the human centrosomal protein CAP350, responsible for FOP recruitment at the centrosome [16] . In addition, TRM1 was shown to target TON1 to the cortical microtubules [15] . FASS encodes a putative protein phosphatase 2A (PP2A) regulatory B′′ subunit [10] , [12] similar to RSA-1, a Caenorhabditis elegans centrosomal protein controlling microtubule outgrowth during spindle formation [17] . PP2As are major eukaryotic phosphatases involved in nearly every cellular process [18] . They comprise a catalytic C subunit, a scaffolding A subunit and a regulatory B subunit, which controls substrate selectivity and subcellular localization of the enzyme [18] . FASS directly interacts with the Arabidopsis PP2AA1/RCN1 subunit [10] , suggesting that it is a genuine subunit of a PP2A complex. Here, we identify a regulatory complex composed of TON1, TRM and a PP2A holoenzyme containing FASS as regulatory subunit using a proteomics approach. We show that the activity of this complex, named TTP (for TON1/TRM/PP2A), is required for PPB formation and spatial control of cell division in land plants. TON1 and FASS form a phosphatase 2A complex in Arabidopsis To gain insight into the protein network involving TON1 and FASS, we performed a series of tandem affinity purifications (TAP) from Arabidopsis suspension cells, using either TON1 (isoforms TON1a and TON1b) or FASS as baits, fused to the GS-tag [19] , [20] . On one hand, complex purifications were performed on cell extracts made in homogenization buffer (HB) with a standard low detergent concentration (0.1% (v/v) Nonidet P-40 (NP-40)) for extraction of water-soluble proteins. On the other hand, complex purifications were performed on extracts made in HB with high detergent concentration (1% (v/v) digitonin) for extraction of both water-soluble and membrane-associated proteins. Both extraction procedures gave comparable results. Moreover, in a total of 30 TAP purifications, only 17 different proteins were specifically and repeatedly co-purified ( Fig. 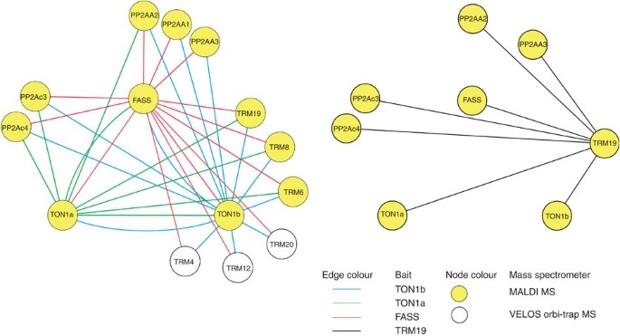Figure 1: TON1 and FASS form a phosphatase 2A complex. TTP protein–protein interaction networks on the basis of the TAP experiments. The left part corresponds to TAP results using TON1a, TON1b or FASS as bait, and the right network corresponds to reverse-TAP experiments using TRM19 as bait protein. Each line represents an interaction in TAP and colours indicate the tagged protein used as bait. White nodes represent the additional interactions identified using the more sensitive VELOS orbitrap analysis. 1 and Table 1 ), indicating the consistency of the TAP approach. Using FASS as bait, we repeatedly identified not only TON1a and TON1b but also PP2A catalytic subunits (PP2AC3/C4), and all three PP2A-scaffolding subunits present in Arabidopsis (PP2AA1/RCN1, PP2AA2 and PP2AA3) ( Fig. 1 , Table 1 , Supplementary Fig. S1 and Supplementary Tables S1–S3 ), showing that FASS is part of a PP2A complex in vivo . Conversely, these PP2A subunits, including FASS, were retrieved with both TON1a and TON1b as baits, confirming that all these proteins are core components of a multi-protein complex ( Fig. 1 and Table 1 ). Interestingly, TAP experiments with TON1a identified TON1b and vice versa , indicating that these proteins likely form heterodimers, presumably via their LisH dimerization domain [11] , [21] . Figure 1: TON1 and FASS form a phosphatase 2A complex. TTP protein–protein interaction networks on the basis of the TAP experiments. The left part corresponds to TAP results using TON1a, TON1b or FASS as bait, and the right network corresponds to reverse-TAP experiments using TRM19 as bait protein. Each line represents an interaction in TAP and colours indicate the tagged protein used as bait. White nodes represent the additional interactions identified using the more sensitive VELOS orbitrap analysis. Full size image Table 1 Summary of tandem affinity purification experiments. Full size table Furthermore, six members from the recently identified TRM protein superfamily [15] were retrieved using TON1a, TON1b and FASS as baits ( Fig. 1 and Table 1 ). Reverse-TAP using the TRM19 GS-tagged protein confirmed co-purification with TON1a and b, FASS and other PP2A subunits ( Fig. 1 and Table 1 ), thereby linking the TON1/FASS-PP2A complex to the TRM family of proteins. Reverse transcriptase PCR (RT–PCR) analyses and available microarray data showed that all five PP2A catalytic subunits are expressed at comparable levels in our suspension cells ( Supplementary Fig. S1a,b ), yet we identified only the closely related isoforms PP2AC3 and C4 in TAP experiments. This likely reflects their preferential incorporation into the TTP complex. On the contrary, over-representation of TRM19 with respect to other TRMs coincides with a high expression level in our cell culture ( Supplementary Fig. S1b ). However, we also retrieved much lower expressors, such as TRM4 or TRM6, confirming that co-purification of a specific isoform does not merely reflects its abundance in our cell system. These results suggest the existence of a high combinatorial diversity of TTP complexes: apart from FASS, all other identified components come into several isoforms, including TON1 (a and b), PP2AC (C3 and C4), PP2AA (A1, A2, A3), as well as a large variety of TRM family members. Several PP2AA and PP2AC isoforms contribute to TTP activity The Arabidopsis genome encodes three PP2AA-scaffolding subunits. PP2AA1 is considered to have a cardinal role in seedlings. Although morphologically similar to the wild type, PP2AA1 mutants display abnormal ethylene and ABA responses, as well as perturbed polar auxin transport [22] , [23] , [24] , [25] . PP2AA2 and PP2AA3 functions are unmasked only in a pp2aa1 mutant background [25] and neither pp2aa2 and pp2aa3 mutant nor pp2aa2-a3 double mutant plants have altered morphological phenotypes per se (see ref. 25 and Fig. 2a ). To analyse genetic interactions between PP2AA genes and FASS , we crossed a weak allele of fass ( fass-14 ) with various pp2aa mutants. Introducing a pp2aa1 mutation in a weak fass background resulted in a much stronger fass phenotype, with a clear gene dosage effect: in a fass-14 background, a heterozygous pp2aa1 mutation significantly enhanced the severity of the fass phenotype, and at the homozygous state the weak fass phenotype was fully converted to a loss-of-function fass phenotype ( Fig. 2b ). Although less marked, a similar enhancer effect was noted when pp2aa2 and pp2aa3 mutations were introduced in a fass-14 background, confirming that all three PP2AA subunits can associate with FASS in vivo ( Fig. 2c ). 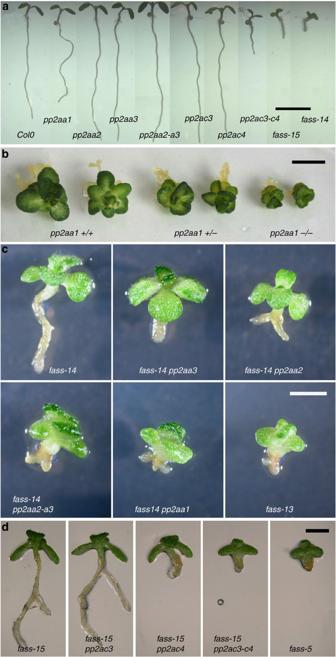Figure 2: Mutations in PP2AA and PP2AC subunits enhance the phenotype of weak fass alleles. (a) Photographs of all crossing partners 6 days after germination. From left to right: wild type (Col0),pp2aa(pp2aa1,pp2aa2,pp2aa3,pp2aa2-a3),pp2ac(pp2ac3,pp2ac4,pp2ac3-c4) andfass(fass-14,fass-15) mutants. (b) Dose-dependent enhancement of thefassphenotype upon introducing aPP2AA1mutation into a weakfass-14mutant background:fass-14seedlings heterozygous for thePP2AA1mutation (middle) already exhibit an enhancedfassphenotype compared with thefass-14line (left), whereaspp2aa1homozygotes (right) show an even more severefassphenotype. (c) Genetic interaction betweenFASSandPP2AAsubunits. CombiningPP2AAmutations with thefass-14allele enhanced thefassphenotype, independent of the A subunit considered. The strongest enhancer effect is obtained with thepp2aa1mutation, aspp2aa1 fass-14double mutant plantlets are indistinguishable fromfassnull ones (fass-13). Mutating eitherpp2aa2, pp2aa3or both significantly increased the severity of the phenotype, although no full conversion to a loss-of-function phenotype was seen in this case. (d) Genetic interaction betweenFASSandPP2ACsubunits. Introducing either thepp2ac3, pp2ac4mutations or both into thefass-15weak allele enhanced thefassphenotype as well, thepp2ac3-c4 fass-15triple mutant being indistinguishable from thefass-5null allele. Scale bars, 1 cm (a); 2 mm (b–d). Figure 2: Mutations in PP2AA and PP2AC subunits enhance the phenotype of weak fass alleles. ( a ) Photographs of all crossing partners 6 days after germination. From left to right: wild type (Col0), pp2aa ( pp2aa1 , pp2aa2 , pp2aa3 , pp2aa2-a3 ), pp2ac ( pp2ac3 , pp2ac4 , pp2ac3-c4 ) and fass ( fass-14 , fass-15 ) mutants. ( b ) Dose-dependent enhancement of the fass phenotype upon introducing a PP2AA1 mutation into a weak fass-14 mutant background: fass-14 seedlings heterozygous for the PP2AA1 mutation (middle) already exhibit an enhanced fass phenotype compared with the fass-14 line (left), whereas pp2aa1 homozygotes (right) show an even more severe fass phenotype. ( c ) Genetic interaction between FASS and PP2AA subunits. Combining PP2AA mutations with the fass-14 allele enhanced the fass phenotype, independent of the A subunit considered. The strongest enhancer effect is obtained with the pp2aa1 mutation, as pp2aa1 fass-14 double mutant plantlets are indistinguishable from fass null ones ( fass-13) . Mutating either pp2aa2, pp2aa3 or both significantly increased the severity of the phenotype, although no full conversion to a loss-of-function phenotype was seen in this case. ( d ) Genetic interaction between FASS and PP2AC subunits. Introducing either the pp2ac3, pp2ac4 mutations or both into the fass-15 weak allele enhanced the fass phenotype as well, the pp2ac3-c4 fass-15 triple mutant being indistinguishable from the fass-5 null allele. Scale bars, 1 cm ( a ); 2 mm ( b – d ). Full size image Likewise, to investigate genetic interactions between FASS and catalytic subunits isolated in our TAP experiments, we introduced pp2ac3 and pp2ac4 mutations into a weak fass-15 mutant background ( Fig. 2d ). The PP2AC3 mutation is expected to be leaky since residual PP2AC3 transcripts are still detectable. Single pp2ac3 or pp2ac4 mutants do not display significant morphological alterations, but pp2ac3-c4 double mutant are dwarfed with thick leaves, flowering stems and siliques ( Fig. 2a and Supplementary Fig. S2 ). When introduced into a fass-15 background, the pp2ac4 mutation induced a strong reduction in root growth as compared with the fass-15 parental seedlings ( Fig. 2d ). pp2ac3-c4 fass-15 triple mutants are even more severely affected and strongly resemble a fass null allele. Depleting scaffolding and catalytic PP2A subunits thus enhance a weak fass phenotype, confirming our physical interaction data, and providing genetic evidence that FASS is part of a bona fide PP2A complex in planta , requiring A1 A2 A3, C3 C4 for full activity. A network of binary interactions establishes the TTP complex The co-purification of FASS, TON1, PP2A and TRM indicated that these proteins are bridged in vivo by physical contacts strong enough to survive the purification procedure. We set up yeast two-hybrid and/or Bimolecular Fluorescence complementation (BiFC) experiments to clarify binary interactions occurring within this large protein complex. TON1 was previously shown to interact with TRM proteins in vivo via the M2 C-terminal motif of the TRMs [15] . BiFC assays revealed that TON1 and FASS interact in Nicotiana cells ( Fig. 3b ). Yeast two-hybrid assays localized this interaction to N-terminal parts of both proteins ( Fig. 3a ). Furthermore, FASS and some TRMs are also capable of interaction: from a two-hybrid screen using FASS as bait, we indeed recovered two TRM clones. One encoded the full-length TRM29, while the other corresponded to the C-terminal part of TRM3 ( Fig. 3c ). To identify the regions responsible for interaction with FASS, we performed two-hybrid assays between FASS and a series of TRM1 deletion fragments. These experiments identified a 110-residue fragment (587–698) sufficient for interaction with FASS ( Fig. 3c ). As TRM1 587–698 , TRM29 and TRM3 645–978 all have the M3 motif in common, the latter likely represents the TRM–FASS interaction region ( Fig. 3c ). 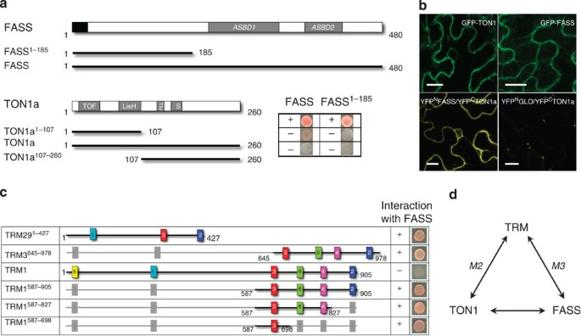Figure 3: FASS interacts with both TON1 and TRMs. (a,b) Interaction between TON1 and FASS. FASS interacts with TON1 in yeast two-hybrid experiments (a) and BiFC experiments inNicotiana benthamianaabaxial epidermal leaf cells (b). (a) Full-length, N- or C-terminal fragments of FASS and TON1 were tested for interaction in yeast two-hybrid. (+) and (−) indicates positive and negative results. Absence of interaction between TON1 full-length protein and FASS might result from improper folding in yeast or from the full-length protein being locked into a ‘closed’ conformation, masking potential interaction domains. Interactions with FASS186–480were meaningless due to strong self-activation of this construct. The position of the two A subunit-binding domains of FASS (ASBD1 and ASBD2) and the TOF, LisH-PLL, and the serine-rich (S) domains of TON1 are indicated. TON1 fragments were fused to the GAL4 activation domain and FASS to the LEX-binding domain. (b) Transient expression assays inNicotiana benthamianaleaf epidermal cells. When overexpressed in this system, GFP-TON1 and GFP-FASS accumulate in the cytoplasm, which is restricted to the cell’s periphery in these epidermal jigsaw puzzle cells. Co-expression of BiFC constructs YFPN-FASS and YFPC-TON1 gave a clear cytoplasmic YFP fluorescence signal, revealing interaction between FASS and TON1. Negative controls correspond to co-expression of YFPC-TON1 with the unrelated YFPN-GLOBOSA protein11(YFPN-GLO). Scale bars, 20μm. (c) The M3 motif of TRMs is involved in direct interaction between TRMs and FASS. A schematic representation of TRMs fragments tested for interaction with FASS in yeast two-hybrid is shown. Coloured boxes correspond to the position of the motifs present in the TRM proteins. (+) and (−) indicates positive and negative results. (d) Schematic view of the interactions between TON1, FASS and TRM proteins. The M2 and M3 motifs of TRMs are involved in interaction with TON1 and FASS, respectively. Figure 3: FASS interacts with both TON1 and TRMs. ( a , b ) Interaction between TON1 and FASS. FASS interacts with TON1 in yeast two-hybrid experiments ( a ) and BiFC experiments in Nicotiana benthamiana abaxial epidermal leaf cells ( b ). ( a ) Full-length, N- or C-terminal fragments of FASS and TON1 were tested for interaction in yeast two-hybrid. (+) and (−) indicates positive and negative results. Absence of interaction between TON1 full-length protein and FASS might result from improper folding in yeast or from the full-length protein being locked into a ‘closed’ conformation, masking potential interaction domains. Interactions with FASS 186–480 were meaningless due to strong self-activation of this construct. The position of the two A subunit-binding domains of FASS (ASBD1 and ASBD2) and the TOF, LisH-PLL, and the serine-rich (S) domains of TON1 are indicated. TON1 fragments were fused to the GAL4 activation domain and FASS to the LEX-binding domain. ( b ) Transient expression assays in Nicotiana benthamiana leaf epidermal cells. When overexpressed in this system, GFP-TON1 and GFP-FASS accumulate in the cytoplasm, which is restricted to the cell’s periphery in these epidermal jigsaw puzzle cells. Co-expression of BiFC constructs YFP N -FASS and YFP C -TON1 gave a clear cytoplasmic YFP fluorescence signal, revealing interaction between FASS and TON1. Negative controls correspond to co-expression of YFP C -TON1 with the unrelated YFP N -GLOBOSA protein [11] (YFP N -GLO). Scale bars, 20μm. ( c ) The M3 motif of TRMs is involved in direct interaction between TRMs and FASS. A schematic representation of TRMs fragments tested for interaction with FASS in yeast two-hybrid is shown. Coloured boxes correspond to the position of the motifs present in the TRM proteins. (+) and (−) indicates positive and negative results. ( d ) Schematic view of the interactions between TON1, FASS and TRM proteins. The M2 and M3 motifs of TRMs are involved in interaction with TON1 and FASS, respectively. Full size image Together with previously published data [15] , this demonstrates that triangular interactions between TRM, FASS and TON1 occur within the TTP complex ( Fig. 3d ), the M2 motif being responsible for the TRM–TON1 interaction, whereas the M3 motif is required for the TRM–FASS interaction. FASS itself is able to form a heterotrimeric PP2A enzyme with A- and C-type subunits. The core TTP is thus composed of at least five protein components. TRMs recruit TTP proteins to microtubule arrays TRMs are a large and diverse superfamily of proteins, in which about half of the members are expected to localize to microtubule arrays [15] . We showed previously that TRM1 localized to cortical microtubules and is able to recruit TON1 to microtubules [15] . We therefore tested whether TRM1, an archetypal TRM member, could recruit other TTP components to microtubule arrays by transient co-expression of TTP proteins in Nicotiana leaf cells. The cytosolic GFP-FASS fluorescence ( Fig. 3b ) relocalized to the cortical microtubules ( Fig. 4d ) upon co-expression with RFP-TRM1. In addition, the BiFC signal of YFP N -FASS and YFP C -TON1a constructs also relocalized from the cytoplasm ( Fig. 4a ) to the cortical microtubule array where it co-localized with RFP-TRM1 ( Fig. 4e ) upon co-expression of the latter. TRM1 was also able to recruit the PP2AA1 subunit complexed with FASS to the microtubules ( Fig. 4f ). Hence, TRM proteins have the ability to recruit not only FASS and TON1 but also other PP2A subunits to microtubule arrays through their interaction with FASS. TRM8 [15] also had the ability to recruit the TON1-FASS BiFC fluorescence to microtubule arrays ( Fig. 4g ), suggesting that microtubule recruitment of TTP proteins is a general function of microtubule-associated TRM proteins. 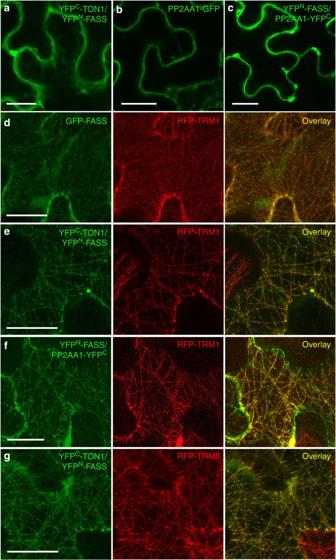Figure 4: TRM proteins target TTP proteins to the microtubular cytoskeleton. (a–c) TON1-FASS (a) and FASS-PP2AA1 (c) BiFC signals, as well as PP2AA1-GFP (b) fluorescence all localized to the cytoplasm when expressed inN. benthamianaleaf epidermal cells. (d–f) Upon co-expression with RFP-TRM1, which labels the cortical microtubular cytoskeletal array (middle panels, red), the GFP-FASS signal (d), the BiFC TON1-FASS fluorescence (e) or the BiFC FASS-PP2AA1 fluorescence (f) relocalized to microtubule arrays where it co-localized as a punctuate staining with TRM1. (g) The BiFC TON1-FASS fluorescence also relocalized to microtubule arrays upon co-expression with RFP-TRM8. All micrographs are projections of Z-stack confocal images. Scale bars, 20 μm (a–g). Figure 4: TRM proteins target TTP proteins to the microtubular cytoskeleton. ( a – c ) TON1-FASS ( a ) and FASS-PP2AA1 ( c ) BiFC signals, as well as PP2AA1-GFP ( b ) fluorescence all localized to the cytoplasm when expressed in N. benthamiana leaf epidermal cells. ( d – f ) Upon co-expression with RFP-TRM1, which labels the cortical microtubular cytoskeletal array (middle panels, red), the GFP-FASS signal ( d ), the BiFC TON1-FASS fluorescence ( e ) or the BiFC FASS-PP2AA1 fluorescence ( f ) relocalized to microtubule arrays where it co-localized as a punctuate staining with TRM1. ( g ) The BiFC TON1-FASS fluorescence also relocalized to microtubule arrays upon co-expression with RFP-TRM8. All micrographs are projections of Z-stack confocal images. Scale bars, 20 μm ( a – g ). Full size image TON1 and FASS together with PP2AA1 decorate the PPB Arabidopsis TON1 and FASS proteins have been shown previously to localize to the PPB [11] , [12] . In addition to a PPB localization, DCD1 and ADD1, the two maize homologues of FASS, persist at the cortical division site after PPB disassembly [13] . To see whether this occurs in Arabidopsis for TON1 and FASS, we studied the dynamic localization of TON1 and FASS during mitosis, using functional GFP-TON1 (ref. 11 ) and GFP-FASS fusions ( Supplementary Fig. S3 ) in root tip cells co-expressing an H2AX-RFP histone marker allowing to precisely define the mitotic phases [26] . Time-lapse imaging of dividing cells showed that both GFP-TON1 and GFP-FASS labelled the PPB and persisted at the cortex up to metaphase, well after PPB disassembly ( Fig. 5a ). We could also show the presence of PP2AA subunits at the PPB by introducing a YFP-PP2AA1 construct [27] in an mCherry-β-tubulin6 background [28] . In root tip cells, YFP-PP2AA1 displayed a cytoplasmic and perinuclear localization as reported before [27] . In addition to this ubiquitous subcellular localization, YFP-PP2AA1 fluorescence distribution along the cortex in cells at the preprophase stage, showed a twofold enrichment at the PPB site ( Fig. 5c ), suggesting association of the PP2AA1 subunit with this structure. 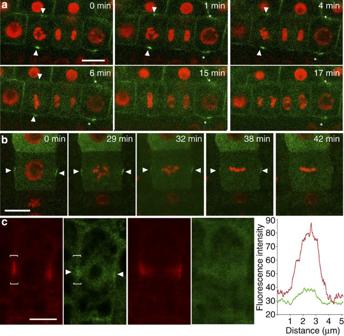Figure 5: TON1 and FASS and PP2AA1 all localize to the PPB. (a) Time-lapse analysis of root tip cells expressing both Pro35S:GFP-FASS and H2AX-RFP showed accumulation of FASS at the cortical division zone during PPB formation, and persistence of the signal beyond PPB degradation up to the metaphase stage. H2AX-RFP served as marker for the different cell-cycle phases. Arrowheads indicate PPB and cortical division zone localization of FASS up to metaphase in cell #1. Note persistence of the signal in cell #2 att=17 min (asterisks), excluding photobleaching-based disappearance of GFP-FASS signal in cell #1. (b) Time-lapse analysis of a root tip cell expressing both Pro35S:GFP-TON1 and H2AX-RFP, showing accumulation of TON1 at the PPB and persistence of the signal at the cortical division zone up to metaphase well after PPB disassembly. (c) Transverse (left) and tangential (right) views of a root tip cell at the preprophase stage expressing ProPP2AA1:YFP-PP2AA1 (green)27and mCherry-β-tubulin6 (red). YFP-PP2AA1 is enriched at the PPB (arrowheads) as also evidenced by the measurement of the fluorescence intensity along the plasma membrane indicated by brackets in transverse views (green curve corresponds to the YFP-PP2AA1 fluorescence and red curve to the mCherry-β-tubulin6 signal). Scale bars, 10 μm (a–c). Figure 5: TON1 and FASS and PP2AA1 all localize to the PPB. ( a ) Time-lapse analysis of root tip cells expressing both Pro35S:GFP-FASS and H2AX-RFP showed accumulation of FASS at the cortical division zone during PPB formation, and persistence of the signal beyond PPB degradation up to the metaphase stage. H2AX-RFP served as marker for the different cell-cycle phases. Arrowheads indicate PPB and cortical division zone localization of FASS up to metaphase in cell #1. Note persistence of the signal in cell #2 at t =17 min (asterisks), excluding photobleaching-based disappearance of GFP-FASS signal in cell #1. ( b ) Time-lapse analysis of a root tip cell expressing both Pro35S:GFP-TON1 and H2AX-RFP, showing accumulation of TON1 at the PPB and persistence of the signal at the cortical division zone up to metaphase well after PPB disassembly. ( c ) Transverse (left) and tangential (right) views of a root tip cell at the preprophase stage expressing ProPP2AA1:YFP-PP2AA1 (green) [27] and mCherry-β-tubulin6 (red). YFP-PP2AA1 is enriched at the PPB (arrowheads) as also evidenced by the measurement of the fluorescence intensity along the plasma membrane indicated by brackets in transverse views (green curve corresponds to the YFP-PP2AA1 fluorescence and red curve to the mCherry-β-tubulin6 signal). Scale bars, 10 μm ( a – c ). Full size image TTP mutants are impaired in division plane positioning Young plantlets of TTP mutant lines exhibit a gradation of a common developmental syndrome, from the strong ton1/fass loss-of-function phenotype to less-affected fass weak mutants, pp2aa1-a2 or pp2aa1-a3 double mutants ( Fig. 6a ), and to a lesser extent pp2ac3-c4 seedlings, likely due to leakiness of the available pp2ac3 allele ( Supplementary Fig. S2 ). 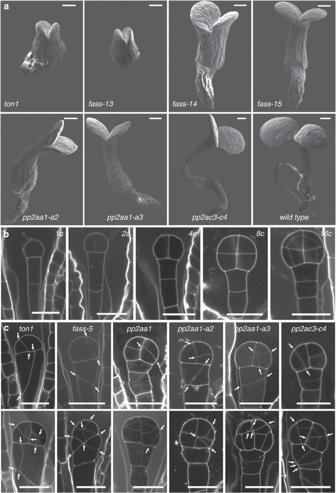Figure 6: TTP mutants share a common developmental syndrome. (a) Scanning electron microscopy images of 3-day-old seedlings of wild type andton1,fass(fass-13, strong allele;fass-14andfass-15weak alleles),pp2aa, andpp2acmutants. (b) Cleavage pattern in wild-type embryos from the single-celled (1c) to the 16-celled stage embryo (16c). The first division of the apical cell of the embryo is longitudinal, whereas the basal cell divides by transverse divisions leading to the formation of the suspensor. The two-celled embryo then divides longitudinally again, perpendicularly to the previous plane. The four resulting cells then divide by transverse divisions, giving rise to the eight-celled embryo. The next round of division establishes the protoderm cell layer by an asymetric cleavage parallel to the surface, to form the 16-celled embryo. (c) Division plane defects inton1, fass-5, pp2aa1,pp2aa1-a2,pp2aa1-a3,pp2ac3-c4mutant embryos. Two representative embryos are shown for each genotype. Abnormal division plane positioning in mutants occurs both in the suspensor and in the embryo proper (arrows). Scale bars, 250 μm (a); 20 μm (b,c). Figure 6: TTP mutants share a common developmental syndrome. ( a ) Scanning electron microscopy images of 3-day-old seedlings of wild type and ton1 , fass ( fass-13 , strong allele; fass-14 and fass-15 weak alleles), pp2aa , and pp2ac mutants. ( b ) Cleavage pattern in wild-type embryos from the single-celled (1c) to the 16-celled stage embryo (16c). The first division of the apical cell of the embryo is longitudinal, whereas the basal cell divides by transverse divisions leading to the formation of the suspensor. The two-celled embryo then divides longitudinally again, perpendicularly to the previous plane. The four resulting cells then divide by transverse divisions, giving rise to the eight-celled embryo. The next round of division establishes the protoderm cell layer by an asymetric cleavage parallel to the surface, to form the 16-celled embryo. ( c ) Division plane defects in ton1, fass-5, pp2aa1 , pp2aa1-a2 , pp2aa1-a3 , pp2ac3-c4 mutant embryos. Two representative embryos are shown for each genotype. Abnormal division plane positioning in mutants occurs both in the suspensor and in the embryo proper (arrows). Scale bars, 250 μm ( a ); 20 μm ( b , c ). Full size image To trace back the origin of these alterations, we followed the cell division pattern in early embryos of TTP mutants. Early embryogenesis in Arabidopsis involves a well-characterized and invariant pattern of cell divisions ( Fig. 6b ). ton1 and fass embryos displayed abnormal division planes in the suspensor and in the embryo proper as early as the two-celled stage, as reported earlier for fass [8] ( Fig. 6c ). Imaging of double pp2aa1-a2 , pp2aa1-a3 or pp2ac3-c4 mutant embryos also revealed notable defects in division plane orientation ( Fig. 6c ). Even pp2aa1 single mutant embryos displayed abnormal division planes ( Fig. 6c and Supplementary Fig. S4 ). This contrasts with the overall normal morphology of pp2aa1 plants post germination ( Supplementary Fig. S5 ) and suggests that the two other PP2AA subunits might compensate for PP2AA1 disruption at later stages of development. Abnormal division plane positioning is thus a shared syndrome of ton1 , fass, pp2aa and pp2ac mutants, further linking these genes in a functional network required for division plane positioning in plant cells. TTP activity is required for preprophase band formation ton1 and fass mutants are defective in PPB formation [9] , [10] , [11] . To search for similar defects in pp2aa or pp2ac mutant cells, we performed immunolocalization of microtubules in dividing root cells. Counter-staining with an anti-KNOLLE antibody allowed to identify cells in early mitosis, as this mitotic marker accumulates at the trans-Golgi network at G2/M [29] , [30] ( Fig. 7 ). At the preprophase stage, in wild type, 96% of KNOLLE-positive cells displayed a PPB, whereas only 4% did not ( n =71). Strikingly, in pp2aa1-a2 or pp2aa1-a3 double mutant cells, no PPBs were observed. In pp2ac3-ac4 double mutants, a majority of cells at the G2/M transition had no discernable PPB (79%, n =34). At the premitotic stage, pp2aa or pp2ac double mutants showed an increased accumulation of perinuclear microtubules, as already noted for ton1 and fass mutants [9] , [10] , [11] . In contrast, all tested mutants formed spindles and phragmoplasts with frequencies and appearance comparable to wild-type cells ( Fig. 7e and Supplementary Fig. S6 ). 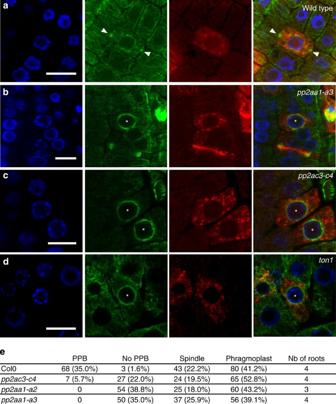Figure 7: pp2aa and pp2ac mutants are impaired in PPB formation. (a–c) Immunolocalizations on root tip cells of 4-day-old seedlings using anti-tubulin (green), DAPI staining (blue) and anti-KNOLLE (red). (a) Wild-type cell at the preprophase stage (PPB marked by the arrowheads) showing KNOLLE accumulation at the trans-Golgi network. (b–d) Absence of PPBs inpp2aa1-a3(b) andpp2ac3-c4(c) double mutants, and in theton1mutant (d). Instead, dense perinuclear microtubules are visible at this stage (asterisks point out the nuclei). Scale bars, 10 μm (a–d). (e) PPB defects inpp2aaandpp2acmutants. Mitotic stages in KNOLLE-positive cells were assessed using the anti-tubulin antibody. The number and percentage of KNOLLE-positive cells with spindles, phragmoplasts, PPBs or without PPB are indicated as well as the number of roots observed. Figure 7: pp2aa and pp2ac mutants are impaired in PPB formation. ( a – c ) Immunolocalizations on root tip cells of 4-day-old seedlings using anti-tubulin (green), DAPI staining (blue) and anti-KNOLLE (red). ( a ) Wild-type cell at the preprophase stage (PPB marked by the arrowheads) showing KNOLLE accumulation at the trans-Golgi network. ( b – d ) Absence of PPBs in pp2aa1-a3 ( b ) and pp2ac3-c4 ( c ) double mutants, and in the ton1 mutant ( d ). Instead, dense perinuclear microtubules are visible at this stage (asterisks point out the nuclei). Scale bars, 10 μm ( a – d ). ( e ) PPB defects in pp2aa and pp2ac mutants. Mitotic stages in KNOLLE-positive cells were assessed using the anti-tubulin antibody. The number and percentage of KNOLLE-positive cells with spindles, phragmoplasts, PPBs or without PPB are indicated as well as the number of roots observed. Full size image In conclusion, defects in PPB formation observed in ton1 , fass and various combinations of PP2A structural and catalytic subunits demonstrate that the TTP-driven PP2A activity is required for PPB formation at the G2/M transition. Since the initial discovery of the PPB almost 50 years ago [31] , numerous studies have confirmed its key role in division plane determination in land plant cells [3] , [7] . However, molecular events contributing to the formation of this fascinating structure are just beginning to be uncovered. TON1 and FASS are among the few identified players in this process, their depletion disorganizing cortical microtubular arrays and preventing PPB formation [8] , [9] , [10] , [11] , [12] . The similar fass and ton1 mutant phenotypes already for long suggested a common mode of action [8] , [9] , [10] , [11] , recently corroborated by the genetic interaction between TON1a and FASS [12] . In this work, we identified a multi-protein complex including TON1, a PP2A heterotrimeric holoenzyme containing FASS as a regulatory subunit, and the TRM proteins. Proteomics, genetics as well as in vivo interaction and recruitment studies contribute to providing a remarkably consistent picture of TTP composition and function in PPB formation. Within the complex, FASS establishes contacts with both TON1 and TRM, which themselves physically interact, in a triangular relationship. These five partners robustly co-purify together and constitute the core of the TTP complex. Co-expression experiments strongly suggest that this complex is recruited to microtubules via the TRM proteins. On the basis of available data, a tentative model emerges, where the PP2A part would represent the enzymatic activity, TON1 an assembly helper and/or activator, and TRM a recruiting agent bringing the PP2A activity into the vicinity of its target(s). Several recent works describe such adaptor proteins targeting PP2A activity to a particular location in the cell (the centrosome [17] and the centromere [32] ) and reveal that PP2A’s specificity is not determined solely by its regulatory B subunits. Therefore, assembly and activation of the whole complex at the proper time and subcellular location establishes specific phosphatase activity playing on the phosphorylation status of protein(s) essential for cortical microtubule dynamics and cytoskeletal transitions. The stoichiometry and dynamics of assembly of core TTP components remains to be established. Our current data show that the core TTP is composed of at least five protein components, for a total MW of ~300 kDa, as also indicated by Blue NativePAGE analysis on cell extracts from cultures expressing GS-tagged TON1a and TON1b ( Supplementary Fig. S1d,e ). However, the diversity of subunits detected in our experiments argues for a combinatorial diversity of TTP isoforms. We provide evidence that all three A-type, but presumably only two (PP2AC3 and PP2AC4 subunits) of the five Arabidopsis C-type PP2A subunits take part in the complex, the three other PP2AC subunits indeed representing a distinct clade among the five PP2AC subunits [33] . This is further corroborated by the recently published analysis of a complete knock-out double pp2ac3-c4 mutant whose phenotype is strikingly reminiscent of ton1 or fass mutants [34] . TON1 also comes into two isoforms, and recent data suggest that TON1a and TON1b are not strictly functionally redundant [12] . The most diverse TTP component is the TRM family, counting 34 members in Arabidopsis . TRMs are able to interact with both TON1 and FASS, thanks to their M2 and M3 motif, respectively. All TRM are predicted to possess a M2 motif, but 11 TRMs do not possess a predicted M3 motif, including TRM6 and TRM8. Yet, both are retrieved in TAP experiments using FASS as bait, suggesting that interaction with TON1 alone might be sufficient for incorporation into the TTP complex, or that the TTP complex can simultaneously contain several TRMs. In total, our TAP and yeast two-hybrid experiments identified half of the TRM family members (17 out of 34) as interactors of TON1 and/or FASS ( Supplementary Fig. S7 ). This makes it likely that all TRM proteins are to some extent capable of contributing to a TON1–TRM–PP2A(FASS) complex. Given their variability in sequence, expression profiles and localization [15] , TRMs are likely a key element for targeting TTP activity to specific cell types and/or subcellular localizations. TRMs are not likely amenable to mutant analysis due to the number of family members suggestive of functional redundancy, but for all other TTP components tested, including TON1, FASS, PP2AA and PP2AC, complete or partial depletion leads to defects in PPB formation and misorientation of division planes. Up to now, TON1 and FASS were the only genes whose mutations induced complete absence of PPBs [8] , [9] , [10] , [11] , [12] , and both proteins colocalize at the PPB and cortical division zone. Here we show that genetic depletion of scaffolding and catalytic PP2A subunits also induces prominent defects in PPB formation and division plane set-up. Although a general reduction in PP2A activity is expected to have pleiotropic effects, it is likely that the PP2A activity specifically associated to the TTP complex is causal to the observed defects. What could be the substrate(s) of such phosphatase activity? An obvious candidate is the TON1 phosphoprotein [35] , which directly interacts and co-localizes with FASS on microtubules, and whose depletion induces the exact same phenotype as the FASS mutation. The TTP complex could also participate in a pathway involved in the regulation of components of the microtubule nucleation machinery, as recent results established a role for FASS in controlling the ratio of in-bundle microtubule nucleation to branched nucleation points [12] . Another potential target is the cortical division zone marker AtTAN, whose persistence at the cortex during preprophase depends on PP2A activity [36] . Several kinases may act to counteract the TTP phosphatase activity since reversible protein phosphorylation/dephosphorylation has an important role in cortical microtubular organization [37] , [38] . One of these could be the cyclin-dependent kinase CDKA;1, previously shown to decorate the late PPB and to induce its disassembly [39] , [40] , [41] , [42] , and which co-purified with TON1 in TAP experiments [43] . Aurora kinases, which in animals are functional antagonists of PP2A at the centrosome and microtubule plus ends [44] , [45] , [46] , are also putative candidates as suggested by recent results pointing to a function for Aurora kinases in premitotic division plane orientation and cortical cytoskeleton organization [47] , [48] . Besides a role in PPB formation, the TTP complex likely has a role in interphase cortical array organization as well. First, the TTP complex is robustly isolated from non-synchronised suspension cells where mitotic cells are a minority. Second, transcription of TTP genes are generally not cell-cycle regulated, with the exception of few TRMs [15] . Furthermore, introducing pp2aa or pp2ac mutations in weak fass alleles that fail to produce PPBs but are still capable of residual interphasic cell elongation, results in a strong fass phenotype and suppresses this residual interphasic growth. Finally, some TRM proteins have been shown to specifically function in cell elongation [15] , [49] . Strikingly, all components of the plant TTP complex identified here show various levels of sequence similarity with animal counterparts localizing transiently or permanently to centrosomes and centrioles/basal bodies. This ranges from whole protein similarity between PP2A subunits (including FASS), to domains conserved between TON1 and FOP, and to conserved motifs between TRM proteins and CAP350 (refs 11 , 16 , 17 ). All available studies point to centrosomal functions for these proteins, either mitotic (RSA1 (ref. 17 )), centrosomal and/or ciliary (FOP/FOR20 (ref. 50 ), CAP350 (ref. 16 )) or linked with cell-cycle progression (FOP [51] ). However, and although animal counterparts of the three core TTP components were recently co-purified in human cells [52] , the function of the TTP network as a whole has not been formally studied in any system apart from plants. The diversity of TRMs in plants, as opposed to the single CAP350 in animals, may reflect the divergence of the two kingdoms with respect to spatial distribution of the nucleation process and organization of the cytoskeleton. Plant material and growth conditions Arabidopsis seedlings were grown on half-strength Murashige and Skoog (MS) medium pH 5.7 containing 1% sucrose (w/v), 0.05% MES (w/v), 0.01% (w/v) myo-inositol and 0.8% agar at 21 °C in a 16-h light/8-h dark regime. The PSB-D Arabidopsis thaliana cell suspension cultures expressing the GS-tag fusion proteins were maintained in 50 ml of MSMO medium (4.43 g l −1 MSMO (Sigma-Aldrich), 30 g l −1 sucrose, 0.5 mg l −1 α-naphthaleneacetic acid, 0.05 mg l −1 kinetin, pH 5.7, adjusted with 1 M KOH) at 25 °C in the dark by gentle agitation (130 r.p.m.). Every 7 days, the cells were subcultured in fresh medium at a 1:6 dilution [43] . Nicotiana benthamiana plants were grown in the growth chamber under 16 h of light, a diurnal temperature of 25 °C and a nocturnal temperature of 20 °C. T-DNA insertion mutants for PP2AC3 (SALK_069250) and PP2AC4 (SALK_035009) were obtained from the Nottingham Arabidopsis Stock Centre [53] . pp2aa mutants were the kind gift of A. Delong [25] . The ton1 mutant carries a deletion affecting both TON1a and TON1b genes [11] . fass mutants in this study have been renamed for clarity: fass-5 , fass-13 , and fass-14 alleles correspond to ton2-5 , ton2-13 and ton2-14 in Camilleri et al. [10] , and fass-15 corresponds to ton2-15 in Kirik et al. [12] Construct design FASS, TON1, PP2AA1, TRM8, TRM1 as well as truncated versions of TON1, TRM1 and FASS open-reading frames were amplified from Arabidopsis complementary DNA clones (Columbia ecotype) using specific primers flanked by AttB1 and AttB2 sites ( Supplementary Table S4 ), cloned into the gateway vector pDONR207 using BP recombination (Invitrogen), and sequenced. Expression vectors were obtained after LR recombination (Invitrogen) between these entry vectors and the following destination vectors: pGWB5 and pGWB6 (ref. 54 ) for expression of C- and N-terminal GFP fusions, respectively, pH7RWG2 and pH7WGR2 (ref. 55 ) for expression of C- and N-terminal RFP fusions, respectively, pBiFP vectors for split YFP experiments [11] , and pLex10- and pGADT7-derived plasmids for yeast two-hybrid interaction assays [15] . Genotyping, RT and qPCR analysis Primers used to genotype pp2aa and pp2ac mutants are indicated in Supplementary Table S4 . Genotyping PCRs were performed on genomic DNA isolated from a rosette leaf [56] . Quantitative PCR (qPCR) and RT–PCR were done on RNA isolated from 6-day-old pp2ac3-c4 double mutant seedlings or RNA from PSB-D cell cultures. RNA was extracted using Trizol (TRI Reagent-Molecular Research Center, Inc.) followed by purification using the RNeasy plant mini kit (Qiagen). cDNA was synthesized from 1 μg of total RNA using the iScript cDNA synthesis kit (Bio-Rad). Five microlitres of ten times diluted cDNA was used for qPCR, performed with the Power SYBR Green mix (Applied Bioscience) on a Roche thermocycler (Roche). Each reaction was done in triplicate and both ACTIN and EIF4A were used as normalization genes. The RT–PCR to analyse the presence of remaining full-length transcript in the pp2ac3-c4 double mutant consisted of 26 repeating cycles with an annealing temperature of 55 °C. The RT–PCR analysis to test for the expression of PP2AA and PP2AC subunits in the PSB-D cell cultures consisted of a touchdown protocol with a gradual decrease of the annealing temperature from 65 to 55 °C during the first 10 cycles followed by 30 cycles with a constant annealing temperature at 55 °C (see Supplementary Table S4 for the primers used). Two-hybrid assays For protein interaction assays, the L40 yeast strain was used ( MATa trp1 leu2 his3 ade2 LYS2::lexA-HIS3 URA3::lexA-lacZ ). Yeast samples transformed with each bait construct (along with empty prey vector) were plated on minimal medium lacking tryptophan, leucine and histidine with increasing concentration of 3-amino-1,2,4-triazole (0–200 mM) to determine the levels of background self-activation of the HIS3 gene. The lowest concentration of 3-amino-1,2,4-triazole that inhibited growth was used to study pairwise interactions in yeast containing both bait and prey vectors. A LexA-FASS fusion protein was used as a bait to screen a custom cDNA library (Invitrogen) prepared from equal amount of Poly-A + RNA of various Col0 Arabidopsis samples (young in vitro -grown seedlings, roots, siliques and seeds, cell-culture suspension, flower buds). Experimental procedures for screening, quantitative β-Gal assays and plasmid isolation were performed according to the manufacturer’s user guide. Plant transformation Overnight Agrobacterium cultures were pelleted, washed and resuspended in infiltration buffer (13 g l −1 S-medium (Duchefa) and 40 g l −1 sucrose, pH 5.7) to an OD600 of 0.5. For co-infiltration experiments, equal volumes of the two (or three or four) cultures of OD 600 of 0.5 were mixed before agro-infiltration. The inoculum was then delivered to the lamina tissue of N. benthamiana leaves by gentle pressure infiltration through the lower epidermis. Negative controls correspond to co-expression of YFP C -TON1 with the unrelated YFP N -GLOBOSA protein, or to co-expression of YFP N -FASS with the unrelated YFP C -DEFICIENS [11] and background levels were checked by expression of YFP C -TON1 or YFP N -FASS alone. Microscopy and immunolocalization For GFP/RFP imaging, fluorescence was recorded using an inverted Zeiss Observer Z1 spectral confocal laser microscope LSM 710 (ref. 15 ). Embryo imaging was performed using propidium iodide staining [57] . Arabidopsis roots of 3- to 4-day-old seedlings were processed for whole-mount immunolocalization [58] using the B-5-1-2 monoclonal anti-α-tubulin (Sigma-Aldrich) and the anti-KNOLLE antibody (kind gift of G. Jürgens). Scanning electron micrographs were obtained using the Hirox SH-1500 microscope with fresh Arabidopsis seedling samples. Tandem affinity purification Transgenes encoding tag fusions were cloned by gateway recombination under control of the constitutive cauliflower tobacco mosaic virus 35S promoter [43] . Transformation of Arabidopsis cell suspension cultures was performed by Agrobacterium co-cultivation and transgenic culture regeneration [43] . TAP of protein complexes was done using the GS tag [19] , [20] with minor buffer modifications for purification in the presence of digitonin: crude protein extracts were obtained with the Ultra-Turrax T25 mixer (IKA Works, Wilmington, NC) using 80% HB without 0.1% (v/v) Nonidet P-40 (NP-40). Afterwards the remaining 20% HB containing 5% digitonin (w/v) was added and the sample incubated for 1 h at 4 °C on a rotating wheel. The cell extract was cleared by two subsequent centrifugation steps at 36,900 × g for 20 min. IgG beads were equilibrated with digitonin-free HB. In both IgG and TEV, wash buffer 0.1% (v/v) NP-40 was replaced by 0.2% (w/v) digitonin. Following TAP, the protein complexes were precipitated and prepared for mass spectrometry analysis. For analysis through MALDI TOF/TOF (TON1a, TON1b, FASS, TRM19, see Supplementary Table S1 for details), proteins were separated by NuPAGE (Invitrogen) [20] . Gel lanes were cut in slices, proteins digested by trypsin and peptides isolated [59] . Mass spectra were obtained by a 4800 MALDI TOF/TOF Proteomics Analyzer (AB SCIEX), and MS-based protein homology identification on the basis of the TAIR genomic database [59] . Experimental background proteins were subtracted on the basis of ~40 TAP experiments on wild-type cultures and cultures expressing TAP-tagged GUS, RFP and GFP mock proteins [59] . For analysis through a LTQ Orbitrap Velos mass spectrometer (Thermo, Bremen, Germany) (TON1a, TON1b and FASS, see Supplementary Methods for details), TCA-precipitated proteins were separated in a short run of 7 min on a 4–12% gradient NuPAGE gel (Invitrogen) and visualized with colloidal Coomassie Brilliant Blue staining. The protein gel was washed for 1 h in H 2 O, polypeptide disulphide bridges were reduced for 40 min in 25 ml of 6.66 mM DTT in 50 mM NH 4 HCO 3 and sequentially the thiol groups were alkylated for 30 min in 25 ml of 55 mM IAM in 50 mM NH 4 HCO 3 . After washing with H 2 O, a broad zone containing the proteins was cut from the protein gel, sliced into 24 gel plugs, and collected together in a single Eppendorf. Gel plugs were washed twice with H 2 O, dehydrated with 95% CH 3 CN (v/v), rehydrated with H 2 O and dehydrated again with 95% CH 3 CN (v/v). Dehydrated gel particles were rehydrated in 60 μl digest buffer containing 750 ng trypsin (MS Gold; Promega, Madison, WI), 50 mM NH 4 HCO 3 and 10% CH 3 CN (v/v) for 30 min at 4 °C. Proteins were digested at 37 °C for 3.5 h. LC-MS/MS runs on LTQ Orbitrap Velos, and peak list generation and submission for protein identification to the TAIR database are described in Supplementary Table S2 (TON1b) and Supplementary Table S3 (TON1a and FASS). Proteins identified with at least two high-confidence peptides were retained. A list of non-specific background proteins was assembled by combining our previous background list [59] with background proteins from control GS purifications on mock, GFP-GS and GUS-GS cell culture extracts and GFP-GS 6-day-old plant extracts identified with Orbitrap VELOS. To obtain the final list of interactors, these background proteins were subtracted from the list of identified proteins. Protein–protein interaction networks were built with the Cytoscape software [60] . Blue Native-SDS–PAGE Total protein extracts from 0.7 g harvested Arabidopsis PSB-D suspension cells expressing 35S::TON1b-GS or 35S::GS-TON1a were prepared according to the NativePAGE Novex Bis-Tris gels electrophoresis protocol by Invitrogen with 0.1% benzonase and 2% digitonin added to the BN lysis buffer. Extracted protein complexes were separated under native conditions over a 4–16% NativePAGE Novex Bis-Tris gel (Invitrogen). Lanes were subsequently cut out and incubated with denaturing buffer (500 mM Tris pH 6.8, 66 mM Na 2 CO 3 , 10% (w/v) glycerol, 2% (w/v) SDS, 2% β-mercaptoethanol) for 1 h under gentle agitation. Denatured first-dimension lanes were placed onto the stacking of a 12% SDS–PAGE gel and the proteins were separated in the second dimension using the Mini-PROTEAN II system (Bio-Rad) for 70 min at 180 V. Proteins in the second-dimension gels were blotted on Immobilon-P membranes (Millipore). Membranes were blocked overnight at 4 °C in 3% (v/v) milk powder dissolved in 25 mM Tris-HCl, pH 8, 150 mM NaCl and 0.1% Triton X-100. Western blots were developed using the Peroxidase Anti-Peroxidase (PAP) antibody (1:2,500) (P1291, Sigma-Aldrich). How to cite this article: Spinner, L. and Gadeyne, A. et al. A protein phosphatase 2A complex spatially controls plant cell division. Nat. Commun. 4:1863 doi: 10.1038/ncomms2831 (2013).